A point mutation inSemaphorin 4Aassociates with defective endosomal sorting and causes retinal degeneration Semaphorin 4A (Sema4A) has an essential role in photoreceptor survival. In humans, mutations in Sema4A are thought to contribute to retinal degenerative diseases. Here we generate a series of knock-in mouse lines with corresponding mutations (D345H, F350C or R713Q) in the Sema4A gene and find that Sema4A F350C causes retinal degeneration phenotypes. The F350C mutation results in abnormal localization of the Sema4A protein, leading to impaired endosomal sorting of molecules indispensable for photoreceptor survival. Additionally, protein structural modelling reveals that the side chain of the 350th amino acid is critical to retain the proper protein conformation. Furthermore, Sema4A gene transfer successfully prevents photoreceptor degeneration in Sema4A F350C/F350C and Sema4A −/− mice. Thus, our findings not only indicate the importance of the Sema4A protein conformation in human and mouse retina homeostasis but also identify a novel therapeutic target for retinal degenerative diseases. The major cause of adult blindness in industrialized countries is the progressive dysfunction and death of retinal photoreceptors. Retinal photoreceptor degeneration is one of the most genetically heterogeneous disorders in humans. Inherited forms of retinal photoreceptor degeneration are defined by their predominantly monogenic inheritance and are a common cause of visual impairment, with a prevalence of ~1 in 3,000 (refs 1 , 2 ). Although many genes have been linked to a photoreceptor degenerative disease phenotype, the mechanisms by which most of these genes lead to this disorder are not fully understood. Semaphorins were initially identified as axonal guidance cues that determine the direction and migration of neurons during neurogenesis [3] . In addition, accumulating evidence has shown that semaphorins have diverse functions in other physiological and pathogenic processes, including vascular development [4] , tumour progression [5] , heart development [6] and immune responses [7] , [8] . Semaphorin 4A (Sema4A) is a class IV transmembrane-type semaphorin. Previously, Rice et al . [9] reported that inserting a gene-trap vector into intron 11 of the mouse Sema4A gene resulted in the loss of retinal photoreceptors. Consistent with their findings, we recently determined that Sema4A-deficient ( Sema4A −/− ) mice display severe photoreceptor degeneration [10] . Notably, we demonstrated that Sema4A, which is expressed in retinal pigment epithelial (RPE) cells, regulates distinct endosomal sorting pathways that are critical for photoreceptor survival and phototransduction during the transition between daylight and darkness [10] . Thus, Sema4A is thought to be one of the genes responsible for retinal degenerative diseases. In fact, three mutations, D345H (345GAC→CAC; D→H), F350C (350TTT→TGT; F→C) and R713Q (713CGG→CAG; R→Q), in the human Sema4A gene have been reported in patients with retinal degenerative diseases based on sequencing of the Sema4A gene from 190 unrelated patients suffering from a variety of retinal degenerative diseases, including retinitis pigmentosa and cone rod dystrophy [11] . However, it has not been determined whether these mutations are really responsible for retinal degeneration, and if so, how mutations in the Sema4A gene induce pathogenesis. In this report, we generated a series of knock-in mouse lines with mutations (D345H, F350C and R713Q) in the Sema4A gene in order to examine the impact of these mutations on the pathogenesis of retinal degenerative diseases. We found that a single point mutation, F350C, caused severe degeneration in photoreceptor cells. In addition, we determined that the pathogenicity of the F350C mutation is due to severe structural defects and resultant mis-localization of the Sema4A protein in RPE cells, which led to impaired endosomal sorting. Furthermore, we provided evidence that Sema4A is a therapeutic target for retinal degenerative diseases using virus-mediated gene therapy. Sema4A F350C/F350C mice exhibit retinal degeneration We first generated a series of knock-in mouse lines that express wild-type (WT) or mutated Sema4A proteins. As the amino-acid sequence of Sema4A is highly conserved between humans and mice, with the 345th, 350th and 713th amino acids being identical, we constructed four knock-in vectors to generate mice with these respective mutations ( Fig. 1a ). Full-size cDNA fragments of WT Sema4A or mutated Sema4A (D345H, F350C or R713Q) fused to enhanced green fluorescent protein (EGFP) at the carboxy terminus were inserted into exon 2 and exon 3 of the Sema4A gene. This series of homozygous knock-in mice appeared normal at birth, developed normally and were fertile, as it is the case for Sema4A −/− mice. Every mutant protein was expressed in tissues ( Fig. 1b ). 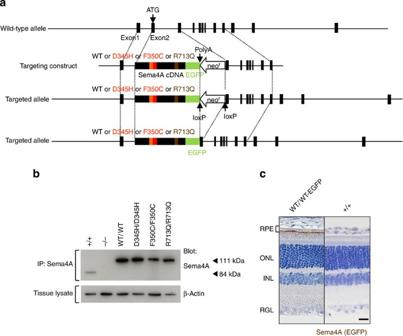Figure 1: Generation of knock-in mice. (a) Schematic diagram of the endogenous mouse locus for theSema4Aknock-in vectors and the resulting Sema4A proteins after homologous recombination. Full-length cDNA fragments of WTSema4Aor mutatedSema4A(D345H, F350C or R713Q) fused with EGFP at the C-terminus were inserted into exon 2 and exon 3 of theSema4Agene. The neomycin resistance gene was flanked by loxP sites so that it could be excised upon expression of Cre recombinase. The gene structure of the WTSema4Aallele (top),Sema4A-targeting construct (second row) and the resultingSema4A-targeted allele in which the neomycin resistance gene was (bottom) or was not (third row) excised. (b) Expression of Sema4A proteins in the brain tissues of knock-in mice. Brain tissues from WT (Sema4A+/+),Sema4AWT/WT,Sema4AD345H/D345H,Sema4AF350C/F350C,Sema4AR713Q/R713QandSema4A−/−(negative control) mice were lysed and subjected to immunoprecipitation (IP) and Western blot analyses using an anti-Sema4A antibody. The 111-kDa bands represent the mutant Sema4A-EGFP proteins (EGFP-tagged), while the 84-kDa band represents the endogenous wild-type Sema4A protein. All series of knock-in mice expressed sufficient amounts of Sema4A protein. (c) Paraffin sections ofSema4AWT/WTor wild-type (Sema4A+/+) (negative control) retinas were examined by immunohistochemistry with an anti-GFP antibody. Sema4A normally localizes at the apical surface of RPE cells in the retina. Scale bar, 50 μm. Figure 1: Generation of knock-in mice. ( a ) Schematic diagram of the endogenous mouse locus for the Sema4A knock-in vectors and the resulting Sema4A proteins after homologous recombination. Full-length cDNA fragments of WT Sema4A or mutated Sema4A (D345H, F350C or R713Q) fused with EGFP at the C-terminus were inserted into exon 2 and exon 3 of the Sema4A gene. The neomycin resistance gene was flanked by loxP sites so that it could be excised upon expression of Cre recombinase. The gene structure of the WT Sema4A allele (top), Sema4A -targeting construct (second row) and the resulting Sema4A -targeted allele in which the neomycin resistance gene was (bottom) or was not (third row) excised. ( b ) Expression of Sema4A proteins in the brain tissues of knock-in mice. Brain tissues from WT ( Sema4A +/+ ), Sema4A WT/WT , Sema4A D345H/D345H , Sema4A F350C/F350C , Sema4A R713Q/R713Q and Sema4A −/− (negative control) mice were lysed and subjected to immunoprecipitation (IP) and Western blot analyses using an anti-Sema4A antibody. The 111-kDa bands represent the mutant Sema4A-EGFP proteins (EGFP-tagged), while the 84-kDa band represents the endogenous wild-type Sema4A protein. All series of knock-in mice expressed sufficient amounts of Sema4A protein. ( c ) Paraffin sections of Sema4A WT/WT or wild-type ( Sema4A +/+ ) (negative control) retinas were examined by immunohistochemistry with an anti-GFP antibody. Sema4A normally localizes at the apical surface of RPE cells in the retina. Scale bar, 50 μm. Full size image Photoreceptor homeostasis is functionally and mechanically supported by RPE cells, which closely interact with photoreceptors via microvilli that interdigitate with the adjacent photoreceptor outer segment. RPE cells perform specialized functions for photoreceptors, including supplying nutrients and factors that protect against light-induced oxidative damage [12] . Immunohistochemistry with an anti-green fluorescent protein (GFP) antibody showed that Sema4A localized at the apical surface of the plasma membrane in RPE cells ( Fig. 1c ), which is consistent with our previous studies [10] . We then examined the histopathology of the respective Sema4A knock-in mice. Of note, only Sema4A F350C/F350C mice exhibited changes in retinal photoreceptors that were compatible with Sema4A −/− mice ( Fig. 2a ). The outer segment of photoreceptors in Sema4A F350C/F350C retina was severely disrupted at 2 weeks of age, followed by a complete loss of photoreceptors at 4 weeks of age ( Supplementary Fig. S1 ). Electroretinography (ERG) monitoring confirmed these histological findings ( Fig. 2b ). A TdT-mediated dUTP nick end labelling (TUNEL) assay demonstrated that Sema4A F350C/F350C retina exhibited a marked increase in the number of apoptotic cells in the outer nuclear layer under illumination ( Fig. 2c ), which was similar to that observed in Sema4A −/− mice [10] . By contrast, Sema4A D345H/D345H and Sema4A R713Q/R713Q mice did not exhibit retinal degeneration ( Fig. 2a ). In addition, Sema4A D345H/+ , Sema4A F350C/+ and Sema4A R713Q/+ mice did not show any retinal defects ( Supplementary Fig. S2 ). Although compound D345H/F350C heterozygous mutations were reported to be associated with retinal degenerative diseases in humans [11] , knock-in mice carrying these mutations did not exhibit this phenotype ( Fig. 2a ). These findings indicate the importance of the 350th amino acid in the function of Sema4A protein. 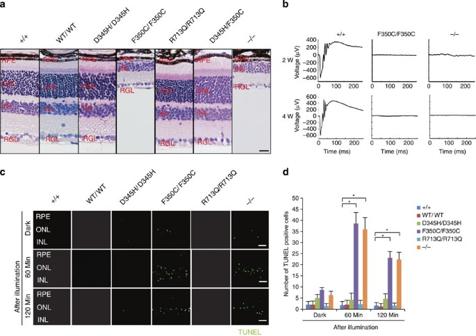Figure 2: Light-induced photoreceptor damage in retinas ofSema4AF350C/F350Cmice. (a) Hematoxylin and eosin (HE) staining of retinas in 4-week-old wild-type (Sema4A+/+),Sema4AWT/WT,Sema4AD345H/D345H,Sema4AF350C/F350C,Sema4AR713Q/R713Q,Sema4AD345H/F350Cand Sema4A-deficient (Sema4A−/−) mice. Among them,Sema4AF350C/F350CandSema4A−/−retinas showed loss of the outer nuclear layer. Scale bar, 50 μm. RPE, retinal pigment epithelium; ONL, outer nuclear layer; INL, inner nuclear layer; RGL, retinal ganglion layer. (b) ERG responses to single flashes were recorded using wild-type (Sema4A+/+),Sema4AF350C/F350CandSema4A−/−mice in a scotopic condition at 2 or 4 weeks of age. Virtually no ERG responses were detected inSema4A−/−andSema4AF350C/F350Cretinas as early as 2 weeks of age. (c) Representative images from the TUNEL assay using P10 mouse retinas after 0, 60 and 120 min of light exposure. Scale bar, 50 μm. (d) Histogram showing the average number of TUNEL-positive cells (±s.e.m.;n=5–10) in retinas. *P<0.01 (Student’st-test). Photoreceptor apoptosis peaked inSema4A−/−andSema4AF350C/F350Cretinas after 60 min of exposure. Data are representative of three independent experiments. Figure 2: Light-induced photoreceptor damage in retinas of Sema4A F350C/F350C mice. ( a ) Hematoxylin and eosin (HE) staining of retinas in 4-week-old wild-type (Sema4A +/+ ), Sema4A WT/WT , Sema4A D345H/D345H , Sema4A F350C/F350C , Sema4A R713Q/R713Q , Sema4A D345H/F350C and Sema4A-deficient ( Sema4A −/− ) mice. Among them, Sema4A F350C/F350C and Sema4A −/− retinas showed loss of the outer nuclear layer. Scale bar, 50 μm. RPE, retinal pigment epithelium; ONL, outer nuclear layer; INL, inner nuclear layer; RGL, retinal ganglion layer. ( b ) ERG responses to single flashes were recorded using wild-type ( Sema4A +/+ ), Sema4A F350C/F350C and Sema4A −/− mice in a scotopic condition at 2 or 4 weeks of age. Virtually no ERG responses were detected in Sema4A −/− and Sema4A F350C/F350C retinas as early as 2 weeks of age. ( c ) Representative images from the TUNEL assay using P10 mouse retinas after 0, 60 and 120 min of light exposure. Scale bar, 50 μm. ( d ) Histogram showing the average number of TUNEL-positive cells (±s.e.m. ; n =5–10) in retinas. * P <0.01 (Student’s t -test). Photoreceptor apoptosis peaked in Sema4A −/− and Sema4A F350C/F350C retinas after 60 min of exposure. Data are representative of three independent experiments. Full size image The Sema4A F350C protein is mis-localized in RPE cells These findings raise the question of why the F350C mutation results in impaired Sema4A functions, even though the expression of this mutant protein is not severely impaired in tissues ( Fig. 1b ). To elucidate this question, we examined protein localization in the retina using the same series of mutant Sema4A knock-in mice. Interestingly, immunohistochemistry revealed that the Sema4A F350C -EGFP protein was abnormally localized. Sema4A F350C -EGFP remained in the cytosol, while Sema4A WT -EGFP, Sema4A D345H -EGFP and Sema4A R713Q -EGFP localized to the surface of RPE cells in the retinas of mutant knock-in mice ( Fig. 3a ) and to the surface of primary cultured RPE cells derived from mutant knock-in mice ( Fig. 3b ). To confirm these findings, we prepared constructs expressing Sema4A WT -EGFP, Sema4A D345H -EGFP, Sema4A F350C -EGFP and Sema4A R713Q -EGFP for in vitro assays, and examined their cellular localization by introducing them into COS-7 cells or a human RPE-derived cell line, ARPE-19 cells. As expected, the Sema4A F350C -EGFP protein failed to reach the plasma membrane, while Sema4A WT -EGFP, Sema4A D345H -EGFP and Sema4A R713Q -EGFP localized to the plasma membrane ( Fig. 3c ). These results indicate that photoreceptor degeneration in Sema4A F350C/F350C mice was due to defects in Sema4A protein localization and distribution in RPE cells. 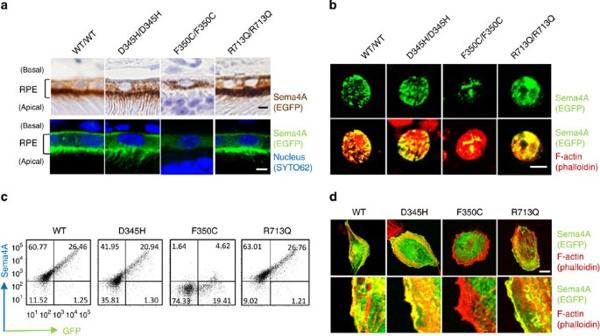Figure 3: The Sema4AF350Cproteins are mis-localized in RPE cells. (a) Representative images of immunostaining of EGFP-tagged Sema4A proteins in RPE cells inSema4AWT/WT,Sema4AD345H/D345H,Sema4AF350C/F350CandSema4AR713Q/R713Qretinas using DAB (top) or fluorescence (bottom). EGFP is shown in brown (top) or green (bottom), and nuclei were visualized with SYTO 62 staining as shown in blue (bottom). Fluorescent signal of EGFP was enhanced by immunostaining using anti-GFP and Alexa Fluor 488-conjugated secondary antibodies (bottom). Scale bar, 2 μm. (b) Immunofluorescent images of primary cultured RPE cells derived fromSema4AWT/WT,Sema4AD345H/D345H,Sema4AF350C/F350CandSema4AR713Q/R713Qmice. EGFP was stained with anti-GFP and Alexa Fluor 488-conjugated secondary antibodies to enhance the GFP signals (green), and the cytoskeleton was visualized by staining with Alexa Fluor 546-conjugated phalloidin as shown in red. Scale bar, 5 μm. (c) Expression of Sema4A on the plasma membrane. COS-7 cells were transfected with plasmid constructs encoding Sema4AWT-EGFP, Sema4AD345H-EGFP, Sema4AF350C-EGFP and Sema4AR713Q-EGFP and incubated for 48 h. Subsequently, the cells were stained with an anti-Sema4A antibody and analysed by flow cytometry. Data are representatives of three experiments. (d) ARPE-19 cells were transfected with plasmid constructs expressing Sema4AWT-EGFP, Sema4AD345H-EGFP, Sema4AF350C-EGFP and Sema4AR713Q-EGFP, incubated for 48 h, fixed, stained with Alexa Fluor 546-conjugated phalloidin, and then examined by confocal microscopy. Representative (top) and enlarged images (bottom) are shown. Scale bar, 10 μm. Figure 3: The Sema4A F350C proteins are mis-localized in RPE cells. ( a ) Representative images of immunostaining of EGFP-tagged Sema4A proteins in RPE cells in Sema4A WT/WT , Sema4A D345H/D345H , Sema4A F350C/F350C and Sema4A R713Q/R713Q retinas using DAB (top) or fluorescence (bottom). EGFP is shown in brown (top) or green (bottom), and nuclei were visualized with SYTO 62 staining as shown in blue (bottom). Fluorescent signal of EGFP was enhanced by immunostaining using anti-GFP and Alexa Fluor 488-conjugated secondary antibodies (bottom). Scale bar, 2 μm. ( b ) Immunofluorescent images of primary cultured RPE cells derived from Sema4A WT/WT , Sema4A D345H/D345H , Sema4A F350C/F350C and Sema4A R713Q/R713Q mice. EGFP was stained with anti-GFP and Alexa Fluor 488-conjugated secondary antibodies to enhance the GFP signals (green), and the cytoskeleton was visualized by staining with Alexa Fluor 546-conjugated phalloidin as shown in red. Scale bar, 5 μm. ( c ) Expression of Sema4A on the plasma membrane. COS-7 cells were transfected with plasmid constructs encoding Sema4A WT -EGFP, Sema4A D345H -EGFP, Sema4A F350C -EGFP and Sema4A R713Q -EGFP and incubated for 48 h. Subsequently, the cells were stained with an anti-Sema4A antibody and analysed by flow cytometry. Data are representatives of three experiments. ( d ) ARPE-19 cells were transfected with plasmid constructs expressing Sema4A WT -EGFP, Sema4A D345H -EGFP, Sema4A F350C -EGFP and Sema4A R713Q -EGFP, incubated for 48 h, fixed, stained with Alexa Fluor 546-conjugated phalloidin, and then examined by confocal microscopy. Representative (top) and enlarged images (bottom) are shown. Scale bar, 10 μm. Full size image In addition, the Sema4A F350C protein did not impair the cell surface expression of the Sema4A WT protein ( Fig. 4a ), indicating that the F350C mutation does not function in a dominant-negative manner. 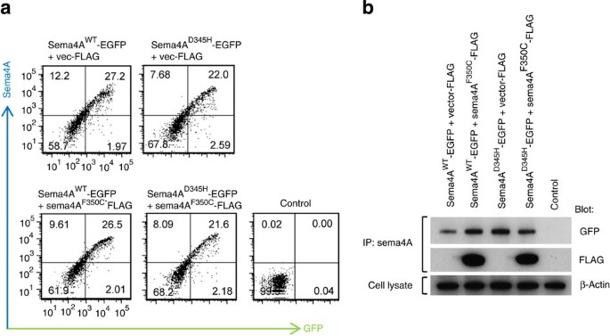Figure 4: Sema4AF350Cprotein does not function in a dominant-negative manner. (a) COS-7 cells were transfected with plasmid constructs encoding Sema4AWT-EGFP, Sema4AD345H-EGFP with or without co-transfection of Sema4AF350C-FLAG. After incubation for 48 h, the cells were stained with an anti-Sema4A antibody and analysed by flow cytometry. Control represents untransfected COS-7 cells with staining in the same conditions. (b) The same transfected COS-7 cells were lysed and subjected to immunoprecipitation (IP) with an anti-Sema4A antibody and subsequent Western blot analyses using anti-GFP (represents Sema4AWT-EGFP or Sema4AD345H-EGFP) or anti-FLAG (represents Sema4AF350C-FLAG) antibodies. Every Sema4A protein was sufficiently expressed in COS-7 cells. Figure 4: Sema4A F350C protein does not function in a dominant-negative manner. ( a ) COS-7 cells were transfected with plasmid constructs encoding Sema4A WT -EGFP, Sema4A D345H -EGFP with or without co-transfection of Sema4A F350C -FLAG. After incubation for 48 h, the cells were stained with an anti-Sema4A antibody and analysed by flow cytometry. Control represents untransfected COS-7 cells with staining in the same conditions. ( b ) The same transfected COS-7 cells were lysed and subjected to immunoprecipitation (IP) with an anti-Sema4A antibody and subsequent Western blot analyses using anti-GFP (represents Sema4A WT -EGFP or Sema4A D345H -EGFP) or anti-FLAG (represents Sema4A F350C -FLAG) antibodies. Every Sema4A protein was sufficiently expressed in COS-7 cells. Full size image The Sema4A F350C protein results in impaired endosomal sorting Moreover, Blue-native PAGE (BN-PAGE) analysis, which separates proteins under native conditions [13] , indicated that the structural integrity of Sema4A was compromised by F350C mutation; the Sema4A F350C protein behaved as high-molecular-weight aggregates on the gel, whereas the other Sema4A proteins migrated as distinct bands corresponding to the monomer and dimer ( Fig. 5a ). In order to explore more about the critical roles of F350 in the Sema4A structure, we prepared a series of Sema4A expression constructs that harbour various mutations in this position, including methionine, tyrosine, glycine and serine (F350M, F350Y, F350G and F350S, respectively). We introduced these expression constructs into ARPE-19 cells or COS-7 cells and examined whether the respective proteins could reach the cell surface. Interestingly, F350M and F350Y, but not F350G and F350S, could reach the plasma membrane ( Fig. 5b ). The result indicates that the mutation is tolerated when F350 is substituted with relatively large amino acids (that is, Met and Tyr), while replacement with small residues (that is, Cys, Gly, and Ser) is detrimental. 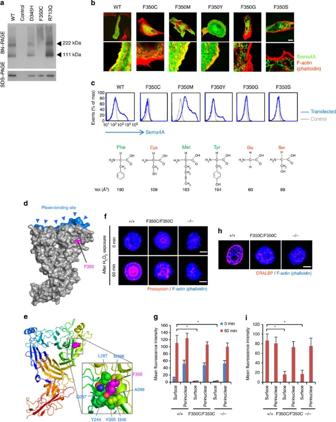Figure 5: The Sema4AF350Cproteins exhibit severe structural defects and impaired function. (a) BN-PAGE and SDS–PAGE with an anti-Sema4A antibody were performed using cell lysates derived from COS-7 cells transfected with constructs expressing Sema4A-EGFP mutant proteins, or pEGFP vector (negative control). In BN-PAGE, the 222-kDa bands represent Sema4A dimers, while the 111-kDa bands represent Sema4A monomers. SDS–PAGE was performed after immunoprecipitation with an anti-Sema4A antibody, using the same lysate as BN-PAGE. (b) Representative images (top) and enlarged images (bottom) obtained by confocal microscopy. ARPE-19 cells were transfected with the plasmid constructs expressing Sema4AF350-EGFP mutant proteins, incubated for 48 h and stained with phalloidin. Scale bar, 10 μm. (c) COS-7 cells were transfected with plasmid constructs and incubated for 48 h, stained with an anti-Sema4A antibody and analysed by flow cytometry. Structural diagrams for amino-acid residue replaced with F350 in each mutant are shown below the histograms, together with their apparent volume per molecule in Å3(ref.34). (d,e) Structural modelling of mouse Sema4A ectodomain, which was built using the structure of human Sema4D structural model previously reported15. (f) Immunofluorescent images of mouse RPE cells after H2O2treatment (250 μM). Prosaposin (red) was peripherally distributed in wild-type (Sema4A+/+) RPE cells but notSema4A−/−orSema4AF350C/F350CRPE cells. Scale bar, 5 μm. (g) Quantitative analysis of the normalized fluorescence intensity of prosaposin at the surface or perinuclear area of the respective RPE cells with (after 60 min) or without (0 min) H2O2treatment (±s.e.m.;n=10). To quantify the intensity, we calculated the mean normalized intensity within the square with its side having an outer 1/6 of radius (‘surface’) or inner 1/6–3/6 of radius (‘perinuclear’). *P<0.01 (Student’st-test). (h) Immunofluorescent images of mouse RPE cells using an anti-CRALBP antibody. Scale bar, 5 μm. (i) Quantitative analysis of the normalized fluorescence intensity of CRALBP on the surface or perinuclear area of RPE cells (±s.e.m.;n=10–15). *P<0.01 (Student’st-test). Figure 5: The Sema4A F350C proteins exhibit severe structural defects and impaired function. ( a ) BN-PAGE and SDS–PAGE with an anti-Sema4A antibody were performed using cell lysates derived from COS-7 cells transfected with constructs expressing Sema4A-EGFP mutant proteins, or pEGFP vector (negative control). In BN-PAGE, the 222-kDa bands represent Sema4A dimers, while the 111-kDa bands represent Sema4A monomers. SDS–PAGE was performed after immunoprecipitation with an anti-Sema4A antibody, using the same lysate as BN-PAGE. ( b ) Representative images (top) and enlarged images (bottom) obtained by confocal microscopy. ARPE-19 cells were transfected with the plasmid constructs expressing Sema4A F350 -EGFP mutant proteins, incubated for 48 h and stained with phalloidin. Scale bar, 10 μm. ( c ) COS-7 cells were transfected with plasmid constructs and incubated for 48 h, stained with an anti-Sema4A antibody and analysed by flow cytometry. Structural diagrams for amino-acid residue replaced with F350 in each mutant are shown below the histograms, together with their apparent volume per molecule in Å 3 (ref. 34 ). ( d , e ) Structural modelling of mouse Sema4A ectodomain, which was built using the structure of human Sema4D structural model previously reported [15] . ( f ) Immunofluorescent images of mouse RPE cells after H 2 O 2 treatment (250 μM). Prosaposin (red) was peripherally distributed in wild-type ( Sema4A +/+ ) RPE cells but not Sema4A −/− or Sema4A F350C/F350C RPE cells. Scale bar, 5 μm. ( g ) Quantitative analysis of the normalized fluorescence intensity of prosaposin at the surface or perinuclear area of the respective RPE cells with (after 60 min) or without (0 min) H 2 O 2 treatment (±s.e.m. ; n =10). To quantify the intensity, we calculated the mean normalized intensity within the square with its side having an outer 1/6 of radius (‘surface’) or inner 1/6–3/6 of radius (‘perinuclear’). * P <0.01 (Student’s t -test). ( h ) Immunofluorescent images of mouse RPE cells using an anti-CRALBP antibody. Scale bar, 5 μm. ( i ) Quantitative analysis of the normalized fluorescence intensity of CRALBP on the surface or perinuclear area of RPE cells (±s.e.m. ; n =10–15). * P <0.01 (Student’s t -test). Full size image Recently, the determination of the crystal structures of semaphorin ectodomains, particularly in complex with their cognate plexin receptors, has led to remarkable progress in our understanding of the structural basis for semaphorin function [14] , [15] , [16] , [17] , [18] . To investigate the structural background of the differential effect of each mutation on the function, we built a structural model of mouse Sema4A ectodomain using the structure of human Sema4D fragment as a template (PDB ID: 1OLZ) [15] . In the model, F350 is located far from the predicted plexin-binding surface ( Fig. 5d ), suggesting that the functional defect exhibited by the mutants is not attributable to a specific loss of plexin-binding activity. Closer inspection of the model revealed that the residue is only partially exposed on the protein surface ( Fig. 5d ), with its large aromatic side chain nestled in a pocket created by many hydrophobic residues ( Fig. 5e ). Therefore, mutation of this residue to amino acids with smaller side chain would create significant vacant space in the protein interior, which is known to harm the overall stability of the protein [19] . Thus, our study clearly demonstrated the importance of the correct cellular localization of Sema4A in RPE cells, which can be fundamentally disturbed by the lack of only a few atoms in a critical amino-acid residue. We previously demonstrated that Sema4A exerts a unique function in the retina, namely by regulating the endosomal sorting of molecules that are indispensable for the phototransduction and survival of photoreceptors [10] . Sema4A regulates two distinct endosomal sorting pathways. First, Sema4A sorts prosaposin, an important antiapoptotic factor, to the plasma membrane of RPE cells, where it is subsequently secreted via exosomes. Second, Sema4A sorts retinoid-binding proteins, including cellular retinaldehyde-binding protein (CRALBP), which is involved in the transport of retinoids to photoreceptors during dark adaptation and the retinoid cycle, to the surface of RPE cells. Indeed, similar to Sema4A −/− cells, RPE cells from Sema4A F350C/F350C retinas expressed lower levels of prosaposin in secreted H 2 O 2 -induced exosomes ( Fig. 5f ), indicating that endosomal sorting is impaired in Sema4A F350C/F350C RPE cells as well as Sema4A −/− RPE cells. CRALBP also failed to distribute to the surface of RPE cells ( Fig. 5h ). These results indicate that the endosomal sorting function of Sema4A was severely impaired by the F350C mutation. Sema4A gene transfer prevents retinal degeneration For potential gene therapy, we finally performed lentivirus-mediated Sema4A gene transfer experiments to determine whether this method could prevent retinal photoreceptor degeneration. According to a previously established transfer method for RPE cells [20] , we prepared lentiviral expression constructs for Sema4A WT -FLAG and Sema4A F350C -FLAG. To confirm the expression patterns of these constructs, we transfected 293T cells with each lentiviral construct. As shown in Supplementary Fig. S3 , Sema4A F350C -FLAG did not reach the cell surface. Next, the Sema4A WT -FLAG- or Sema4A F350C -FLAG-expressing lentiviral suspension was injected into the subretinal space of 1-week-old Sema4A −/− or Sema4A F350C/F350C mice using a transvitreous approach ( Fig. 6a ). Three weeks after injection, the eye tissues were fixed and sectioned. In mice injected with lentiviral vectors expressing Sema4A WT -FLAG, the layer of photoreceptor cells was substantially preserved on the injected side alone in both Sema4A −/− and Sema4A F350C/F350C retinas ( Fig. 6b ). In contrast, injecting with lentiviral vectors expressing Sema4A F350C -FLAG did not prevent photoreceptor degeneration in either Sema4A −/− or Sema4A F350C/F350C mice. Immunohistochemistry confirmed that the injection of these lentiviral vectors resulted in sustained expression of the Sema4A WT -FLAG or Sema4A F350C -FLAG proteins specifically in RPE cells ( Fig. 6b ). In addition, injecting lentiviral vectors expressing Sema4A WT -FLAG restored ERG responses to some extent in Sema4A −/− and Sema4A F350C/F350C retinas ( Fig. 6d ). Notably, we observed long-term preservation of the photoreceptor layer, lasting at least 4 months after gene transfer ( Fig. 7 ). Thus, we demonstrated a successful means to prevent retinal photoreceptor degeneration using lentivirus-mediated Sema4A gene transfer. 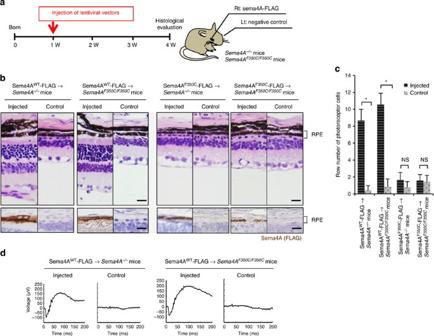Figure 6:Sema4Agene transfer prevents photoreceptor degeneration in the retinas ofSema4A−/−andSema4AF350C/F350Cmice. (a) Schematic diagram of the protocol: At 1 week of age, suspensions of lentiviral vectors expressing Sema4AWT-FLAG or Sema4AF350C-FLAG were injected into the subretinal space ofSema4A−/−orSema4AF350C/F350Cinfant mice. Viral suspensions were injected into the right eye, while the left eye was used as a negative control (only eyelids were incised). At 4 weeks of age, their eye tissues were fixed and sectioned. (b) (Top) Haematoxylin and eosin (HE) staining of the retinal sections from each mouse. Scale bar, 50 μm. (Bottom) The serial sections from those of HE staining were examined by immunohistochemistry (IHC) using an anti-FLAG antibody. Scale bar, 50 μm. (c) Histogram showing the average number of photoreceptor cells (±s.e.m.;n=9–18) in retinas. *P<0.01 (Student’st-test); NS, not significant. The number of row of photoreceptor cells was counted at three random points per retinal section in which Sema4AWT-FLAG or Sema4AF350C-FLAG was expressed in immunohistochemistry using an anti-FLAG antibody. (d) ERG responses to single flashes were recorded usingSema4A−/−orSema4AF350C/F350Cmice afterSema4Agene transfer. A suspension of lentiviral vectors expressing Sema4AWT-FLAG was injected into the retinas ofSema4A−/−orSema4AF350C/F350Cmice at 1 week of age, and ERGs were recorded at 4 weeks of age. Viral suspensions were injected into the right eye, while the left eye was used as a negative control (only eyelids were incised). Figure 6: Sema4A gene transfer prevents photoreceptor degeneration in the retinas of Sema4A −/− and Sema4A F350C/F350C mice. ( a ) Schematic diagram of the protocol: At 1 week of age, suspensions of lentiviral vectors expressing Sema4A WT -FLAG or Sema4A F350C -FLAG were injected into the subretinal space of Sema4A −/− or Sema4A F350C/F350C infant mice. Viral suspensions were injected into the right eye, while the left eye was used as a negative control (only eyelids were incised). At 4 weeks of age, their eye tissues were fixed and sectioned. ( b ) (Top) Haematoxylin and eosin (HE) staining of the retinal sections from each mouse. Scale bar, 50 μm. (Bottom) The serial sections from those of HE staining were examined by immunohistochemistry (IHC) using an anti-FLAG antibody. Scale bar, 50 μm. ( c ) Histogram showing the average number of photoreceptor cells (±s.e.m. ; n =9–18) in retinas. * P <0.01 (Student’s t -test); NS, not significant. The number of row of photoreceptor cells was counted at three random points per retinal section in which Sema4A WT -FLAG or Sema4A F350C -FLAG was expressed in immunohistochemistry using an anti-FLAG antibody. ( d ) ERG responses to single flashes were recorded using Sema4A −/− or Sema4A F350C/F350C mice after Sema4A gene transfer. A suspension of lentiviral vectors expressing Sema4A WT -FLAG was injected into the retinas of Sema4A −/− or Sema4A F350C/F350C mice at 1 week of age, and ERGs were recorded at 4 weeks of age. Viral suspensions were injected into the right eye, while the left eye was used as a negative control (only eyelids were incised). 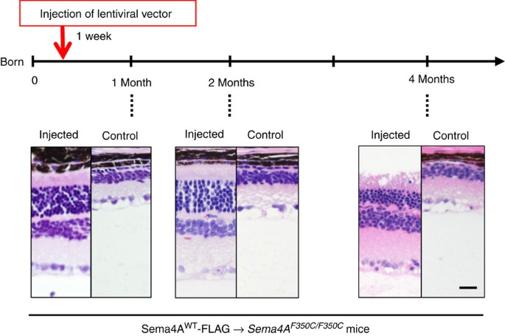Figure 7: Long-term prevention of photoreceptor degeneration afterSema4Agene transfer. Similar toFigure 6, gene transfer with the lentiviral vectors expressing Sema4AWT-FLAG was performed in 1-week-old Sema4AF350C/F350Cmice. Subsequently, we evaluated the retinal histology of these mice at 1, 2 or 4 months of age to estimate the duration of the therapeutic effects. As shown in the representative images, photoreceptor cells were preserved at least 4 months after gene transfer. Scale bar, 50 μm. Full size image Figure 7: Long-term prevention of photoreceptor degeneration after Sema4A gene transfer. Similar to Figure 6 , gene transfer with the lentiviral vectors expressing Sema4A WT -FLAG was performed in 1-week-old Sema4A F350C/F350C mice. Subsequently, we evaluated the retinal histology of these mice at 1, 2 or 4 months of age to estimate the duration of the therapeutic effects. As shown in the representative images, photoreceptor cells were preserved at least 4 months after gene transfer. Scale bar, 50 μm. Full size image Here we highlighted a novel pathogenic trait of retinal degenerative diseases by analysing a series of knock-in mice with Sema4A mutations, which are thought to contribute to human retinal degenerative disease [11] . Among these mice, only Sema4A F350C/F350C mice exhibited light-induced retinal degeneration that occurred immediately after birth, which is similar to that observed in Sema4A −/− mice ( Fig. 2a ). In addition, a protein structural modelling and mutational analysis of the Sema4A protein revealed that the side-chain volume of the 350th amino acid is critical for its proper conformation and function in the endosomal sorting of molecules indispensable for photoreceptor survival ( Fig. 5d–i ). We further determined that Sema4A has therapeutic effects in retinal degenerative diseases using virus-mediated gene therapy ( Fig. 6 ). Recently, we reported that Sema4A mediated the exosomal release of prosaposin and endosomal sorting of retinoid-binding proteins, including CRALBP, in RPE cells [10] . The finding that Sema4A functions as an intracellular guide for specific molecules was highly significant because semaphorins and their receptor plexins were previously shown to function as extracellular guidance molecules [3] . Indeed, our structural modelling of the Sema4A protein indicated that the plexin-binding site is distant from the 350th amino acid ( Fig. 5d ), suggesting that this mutation does not block this ligand–receptor interaction. This notion is consistent with our previous finding that mice lacking Sema4A receptors exhibited no apparent retinal defects [10] . However, as Plexin-D1-deficient mice die soon after birth [21] , we cannot exclude a possibility that the defects are potentially mediated by interacting receptors. Further careful evaluation would be required to determine the pathogenesis. In addition, BN-PAGE analysis showed that the F350C mutation causes intracellular aggregation of the Sema4A protein, probably within the endoplasmic reticulum, in RPE cells ( Fig. 5a ). Thus, it appears that this structural defect prevents the protein from being properly transported to its cellular compartments. In this context, the present findings support the notion that Sema4A can function as an ‘intracellular navigator’ that releases molecules essential for photoreceptor survival. It is also noteworthy that the Sema4A F350C protein did not affect the expression of the Sema4A WT and Sema4A D345H proteins ( Fig. 4 ), indicating that this mutated protein does not function in a dominant-negative manner. Sema4A D345H/D345H and Sema4A R713Q/R713Q mice did not show a disease phenotype in our study ( Fig. 2a ). In our mouse Sema4A ectodomain model, D345 is located in an α-helix with its side chain well exposed to the solvent and R713 is located in the short cytoplasmic tail region, which is unlikely to form a structural domain. Therefore, both D345H and R713Q do not seem to cause major structural destabilization, which is further supported by the normal cell surface expression of these mutants ( Fig. 3a ). However, we cannot completely exclude the possibility that these mutations contribute to the pathogenicity of human retinal degenerative diseases. There are several possibilities for the differences between our study using mutant mice and a previous human study [11] . First, humans have a longer lifespan than mice, and thus F350C heterozygosity (with D345H) in humans may ultimately induce retinal degenerative disease owing to reduced expression of functional Sema4A proteins. Second, we should carefully evaluate the findings of the human study because this report only sequenced the Sema4A gene but did not definitively exclude the possible involvement of other genetic factors. In addition, the human report did not include the phenotypes of F350C homozygotes. Third, slight amino-acid differences between human and mouse Sema4A might contribute to the fragility of the human Sema4A protein structure with a D345H mutation. It has been recently reported that transiently expressed human Sema4A D345H mutant protein showed altered intracellular localization in human RPE cell lines [22] . Additionally, as large-scale sequential analyses of patient DNA have not been performed except for Pakistani individuals [11] , further studies will be required to determine whether patients in other racial groups possess the same mutation. We presented evidence that virus-mediated Sema4A gene transfer was successful in an animal model ( Fig. 6 ). Thus, it is theoretically possible to treat this type of retinal degenerative disease with gene therapy, if performed immediately after birth. Recently, considerable progress has been made in the development of gene therapy for retinal degenerative diseases using recombinant adeno-associated virus or lentivirus-based vectors [23] . Currently, RPE65 , which encodes the retinoid isomerase enzyme and causes Leber congenital amaurosis, is the first and only gene that has been successfully treated by gene transfer therapy in human eyes [24] , [25] , [26] , [27] , [28] , [29] . As Sema4A gene transfer displayed a strong curative effect that was comparable to that of RPE65 at least in the histology in animal models, it appears that Sema4A might be a candidate therapy for retinal degenerative diseases. However, although ERG responses could be detected after gene transfer ( Fig. 6d ), the levels of responses were relatively low compared to those in WT retinas ( Fig. 2b ). Deeper investigations would be necessary to reveal the extent of the gene transfer efficacy. As retinal degenerative diseases are caused by many genetic changes, Sema4A gene therapy might be limited to a subset of patients carrying Sema4A genetic changes, such as the F350C mutation. However, considering the endosomal sorting function of Sema4A for various molecules that are indispensable for retinal homeostasis, it is possible that Sema4A replacement gene therapy might be efficacious in a wider subset of patients with retinal degenerative diseases. Further studies are required to assess the potential of Sema4A gene therapy. Collectively, we demonstrated that Sema4A is required for photoreceptor survival. We determined that a point mutation in the Sema4A gene causes retinal degenerative disease, which was further supported by structural modelling analyses. The F350C mutation reduces the amino-acid side-chain volume and creates a significant vacant space in the protein interior, which is known to affect the overall stability of the protein [19] and may lead to the precipitation of the protein into non-functional aggregates. Furthermore, photoreceptor degeneration could be rescued by Sema4A gene supplementation in an animal model. Our findings provide a novel therapeutic target for retinal degenerative diseases. Animals Sema4A −/− mice (previously established [30] ) as well as all knock-in mice (Sema4A WT/WT mice, Sema4A D345H/D345H mice, Sema4A F350C/F350C mice, Sema4A R713Q/R713Q mice, Sema4A D345H/F350C mice, Sema4A WT/+ mice, Sema4A D345H/+ mice, Sema4A F350C/+ mice and Sema4A R713Q/+ mice) and WT mice (Sema4A +/+ mice) with the same genetic background (C57BL/6J) were housed under a 12-h light/12-h dark cycle (60 lux at the cage level). All animal procedures were performed in accordance with institutional guidelines. Construction of the expression vector and site-directed mutagenesis The cDNA sequence encoding full-length Sema4A (amino acids 1–760) was generated by PCR and then ligated into pEGFP-N3 (Clontech, Palo Alto, CA) or p3xFLAG-CMV-14 (Sigma-Aldrich Co., Milwaukee, WI). Various mutant constructs (Sema4A D345H -EGFP, Sema4A F350C -EGFP, Sema4A R713Q -EGFP, Sema4A F350M -EGFP, Sema4A F350Y -EGFP, Sema4A F350G -EGFP, Sema4A F350S -EGFP and Sema4A F350C -FLAG) were generated from Sema4A WT -EGFP or Sema4A WT -FLAG using a QuikChange II XL site-directed mutagenesis kit (Stratagene, La Jolla, CA) according to the manufacturer’s protocol. Gene targeting strategy DNA fragments were isolated from Sema4A WT -EGFP, Sema4A D345H -EGFP, Sema4A F350C -EGFP and Sema4A R713Q -EGFP constructs. To construct targeting vectors (for Sema4A WT/WT , Sema4A D345H/D345H , Sema4A F350C/F350C and Sema4A R713Q/R713Q mice), the 3.1-kb fragments encoding full-length WT or mutant Sema4A cDNA containing EGFP at the C-terminus were placed into exon 2 and exon 3 in the intact Sema4A alleles. The Herpes simplex virus thymidine kinase ( HSV-tk ) gene was inserted to select against random integration. The linearized targeting plasmid DNA was electroporated into ES cells. After selecting with G418, resistant colonies were screened for homologous recombination of the Sema4A -targeted allele by PCR and Southern blot analysis. The clones with homologous recombination were identified and isolated. These ES cells were injected into blastocysts from C57BL/6J mice. The blastocysts were transferred to pseudopregnant ICR foster mothers, and chimeric males were obtained. Subsequently, chimeric males and WT females were mated to produce heterozygous, targeted mice. Cell culture ARPE-19 cells, COS-7 cells and 293T cells were grown in DMEM supplemented with 10% fetal calf serum. RPE cells were isolated from 10-day-old mice for primary cultures following an experimental procedure that was previously described [31] . Briefly, enucleated eyecups were treated with 2% dispase (Invitrogen, San Diego, CA) and 0.5% trypsin/EDTA (Gibco BRL Life Technologies, Rockville, MD), and the isolated RPE cells were seeded into fibronectin-coated cell culture dishes (BD BioCoat) (BD Bioscience, San Jose, CA) and grown in DMEM containing 10% fetal bovine serum at 37 °C. RPE cells were successfully subcultured using 0.5% trypsin/EDTA every 7 days for 1 month. Immunomethods The antibodies used to detect Sema4A were previously described [30] . The other antibodies used in this study include anti-GFP (Cell Signaling Technology Inc., Danvers, MA), anti-FLAG (Cell Signaling Technology Inc., Danvers, MA), anti-prosaposin (Abcam, Cambridge, UK) and anti-CRALBP (Abcam, Cambridge, UK). Cells were transfected using FuGENE HD (Roche Applied Science, Indianapolis, IN) and then incubated for 2 days, collected and lysed in lysis buffer (50 mM Tris–HCl at pH 8.0, 250 mM NaCl, 5 mM EDTA, 1% NP-40, 0.25% Na-deoxycholate and 1 mM NaF) for immunoprecipitation and immunoblot analyses, which were performed using standard protocols. SDS–polyacrylamide gel electrophoresis (SDS–PAGE) and BN-PAGE For SDS–PAGE, samples were boiled for 5 min in SDS–PAGE sample buffer containing 0.125 mM Tris–HCl, pH 6.8, 20% glycerol, 4% SDS, 10% 2-mercaptoethanol and 0.004% bromophenol blue. The protein samples were loaded onto NuPAGE 4–12% Bis–Tris gels (Invitrogen, San Diego, CA). BN-PAGE systems were purchased from Invitrogen, and sample preparation and electrophoresis were performed according to the manufacturer’s instructions. For immunoblot analysis, the gel was electroblotted onto a PVDF membrane, which was blocked in 5% skim milk and incubated with an anti-Sema4A antibody followed by a goat anti-rabbit secondary antibody. Immunohistochemistry of paraffin-embedded specimens Eyecup specimens were fixed in 4% paraformaldehyde and routinely processed for paraffin embedding. Paraffin-embedded specimens were cut into 4-μm-thick sections and stained using the immunoperoxidase procedure. After antigen retrieval with a Pascal pressurized heating chamber (DAKO A/S, Glostrup, Denmark), the sections were treated with Melanin bleach Kit (Polysciences Inc., Warrington, PA) to remove melanin from RPE cells, incubated with the indicated antibodies and then treated with ChemMate EnVision kit (DAKO A/S, Glostrup, Denmark). DAB (DAKO A/S, Glostrup, Denmark) was used as a chromogen. Immunohistochemistry of frozen specimens Frozen sections of 4% paraformaldehyde-fixed eyecups of 8 μm thickness were prepared. The sections were treated with Melanin bleach Kit (Polysciences Inc., Warrington, PA) to remove melanin from RPE cells, incubated with a blocking solution (5% BSA in PBS containing 0.5% Triton X-100) for 1 h, and then stained overnight with the indicated antibodies. Confocal images were obtained using an LSM 5 EXCITER (Ver 4.2) confocal inverted microscope (Carl Zeiss MicroImaging, Jena, Germany). TUNEL assay TUNEL assay systems (DeadEnd Fluorometric TUNEL system) were purchased from Promega (Madison, WI). Prepared frozen sections were processed according to the manufacturer’s protocol. Sections were imaged using an LSM 5 EXCITER (Ver 4.2) confocal inverted microscope (Carl Zeiss MicroImaging, Jena, Germany). Electroretinography Conventional full-field ERGs were recorded in vivo using a PuREC system with two built-in white LED contact lens electrodes (Mayo, Aichi, Japan). Mice were dark-adapted overnight and all subsequent procedures were performed under dim red light. Before the ERG recordings, mice were anaesthetized and placed on a heating pad held at 37 °C throughout the experiments. The pupils were dilated with a cocktail of 0.05% tropicamide and 0.05% phenylephrine hydrochloride. 0.5% hydroxyethyl cellulose was applied to the eyes to maintain corneal hydration. Needle electrodes placed subcutaneously in the forehead and tail served as reference and ground electrode, respectively. Single-flash recordings were performed at a light intensity of 2.0 log cd s m −2 using a sampling frequency of 1,253 Hz and a flash duration of 13.3 ms. The band-pass filter was set between 0.3 and 500 Hz. In addition, the obtained data were low-pass filtered at 300 Hz using a PuREC software (Mayo, Aichi, Japan). Homology model building Sequence alignments of the ectodomain portions of mouse Sema4A (residues 36–650) and human Sema4D (residues 24–648) were generated using CLUSTALW [32] . Homology model building was performed with the programme MODELLER [33] using the human Sema4D ectodomain structure (PDB ID: 1OLZ) [15] as a template. Preparation of lentiviral vectors C-terminal FLAG-tagged Sema4A cDNA fragments with or without the F350C mutation were isolated and amplified by PCR from the Sema4A WT -p3xFLAG-CMV-14 or Sema4A F350C - p3xFLAG-CMV-14 constructs. The PCR primers contained an Age I site at the 5′-terminus and Eco RI site at the 3′-terminus. Primer sequences are described in Supplementary Table S1 . This fragment was digested with Age I and Eco RI, and subsequently subcloned into the Age I and Eco RI sites of CSII-CMV-MCS (RIKEN, Tokyo, Japan). The titres of the Sema4A WT -FLAG and Sema4A F350C -FLAG lentiviral vectors were determined by quantitative RT-PCR using viral RNA from 293T cells infected with these vectors. After the virus was concentrated by ultracentrifugation, titres of 5 × 10 7 infectious units ml −1 for the Sema4A WT -FLAG lentiviral vector and 1.3 × 10 7 infectious units ml −1 for the Sema4A F350C -FLAG lentiviral vector were obtained. In vivo delivery of lentiviral vectors Infant mice (1 week of age) were anaesthetized. The eyeball was exposed by an incision in the eyelid, parallel to the future edge of the open eyelid. Subretinal injections were performed under an operating microscope. A small incision was made in the sclera, and 2 μl of undiluted vector suspension (titres of 1.3–5 × 10 7 infection units ml −1 on 293T cells) was injected through the incision into the subretinal space using a glass capillary connected to a 10-μl syringe. How to cite this article: Nojima, S. et al . A point mutation in Semaphorin 4A associates with defective endosomal sorting and causes retinal degeneration. Nat. Commun. 4:1406 doi: 10.1038/ncomms2420 (2013).